Enhanced acoustic sensing through wave compression and pressure amplification in anisotropic metamaterials Acoustic sensors play an important role in many areas, such as homeland security, navigation, communication, health care and industry. However, the fundamental pressure detection limit hinders the performance of current acoustic sensing technologies. Here, through analytical, numerical and experimental studies, we show that anisotropic acoustic metamaterials can be designed to have strong wave compression effect that renders direct amplification of pressure fields in metamaterials. This enables a sensing mechanism that can help overcome the detection limit of conventional acoustic sensing systems. We further demonstrate a metamaterial-enhanced acoustic sensing system that achieves more than 20 dB signal-to-noise enhancement (over an order of magnitude enhancement in detection limit). With this system, weak acoustic pulse signals overwhelmed by the noise are successfully recovered. This work opens up new vistas for the development of metamaterial-based acoustic sensors with improved performance and functionalities that are highly desirable for many applications. Acoustic sensors are critically needed for the detection of pressure waves in many applications, including acoustic surveillance [1] , acoustic navigation and communications [2] , structural health monitoring [3] and medical imaging and therapy [4] . Over the last two decades, considerable progress has been made in the development of novel acoustic sensors, including piezoresistive [5] , piezoelectric [6] , capacitive [7] and optical-based sensors [8] , [9] . However, the detection capability of these sensors is fundamentally limited by their minimal detectable pressure. This fundamental limit hinders the performance of many acoustic systems, such as the surveillance range of sonar, data transmission performance of acoustic communications and detection depths and detectable tumour sizes of ultrasonic imaging systems [10] . Therefore, there is still a great need to develop novel sensing modalities and functional materials that can overcome the limitations of current acoustic sensing technologies. Acoustic metamaterials, similar to their electromagnetic counterparts [11] , [12] , [13] , are artificial materials designed to manipulate sound waves [14] . Over the past decade, acoustic metamaterials have been extended far beyond the scope of original negative refraction materials, and metamaterials with large values of positive or negative mass densities, bulk moduli and refractive indices have been demonstrated [15] , [16] , [17] , [18] , [19] , [20] . On the other hand, there have been ever-growing activities in the development of acoustic metamaterial devices, such as metamaterial imaging and lenses systems [21] , [22] , [23] , [24] , [25] , waveguide [26] , invisible cloaking [27] , [28] , [29] , [30] , [31] , sound isolators [32] , [33] , [34] and acoustic absorbers [35] , which have superior performance over their conventional counterparts. It is expected that acoustic metamaterials will continue to offer unprecedented opportunities to advance acoustic technologies. Given the importance of acoustic sensing in many fronts, it is of great interest to explore metamaterial-based acoustic sensing systems that can achieve unparalleled performance and functionalities. Recently, a new class of metamaterials based on strong anisotropic structures has emerged [36] , [37] , [38] . This gives rise to the field of anisotropic metamaterials, which enable flexible control of electromagnetic and acoustic waves for realizing functional devices with unique properties [22] , [23] , [28] , [39] , [40] , [41] . Here we report a metamaterial-enhanced acoustic sensing system based on highly anisotropic acoustic metamaterials (see Fig. 1 ). These materials allow sound propagation with a large wave vector k , rendering a high-refractive-index medium. This means that the wavelength of sound will be shortened, which enables a spatial concentration of wave energy and induces a strong pressure enhancement in the metamaterials. Therefore, enhanced acoustic sensing can be achieved by detecting the significantly amplified pressure field in such high-refractive-index medium. As proof of concept, we demonstrate acoustic wave propagation and compression in one type of highly anisotropic metamaterials, that is, the graded high-refractive-index metamaterials constructed with alternating subwavelength air–metal layers. To understand the wave compression and pressure amplification phenomenon, closed-form analytical expressions are obtained to describe the spatial and spectral pressure field distributions in the metamaterials, which are further validated by using numerical simulations. In our experiments on a prototype metamaterial device, pressure amplification of over an order of magnitude is achieved. By using such a metamaterial device for enhancing acoustic sensing, recovery of time-domain acoustic pulses overwhelmed by the noise floor is successfully demonstrated. 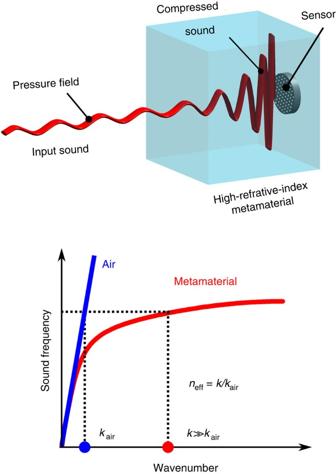Figure 1: Schematic of metamaterial-enhanced acoustic sensing. Top: the pressure field of sound is spatially compressed and amplified inside the high-refractive-index acoustic metamaterial before being detected by a sensor. Bottom: schematic metamaterial dispersion curve for acoustic waves with a high-kstate. In such a metamaterial medium, sound propagation with a large wave vectork(measured by wave number) is enabled, rendering an effective high-refractive-indexneff=kz/kair. Figure 1: Schematic of metamaterial-enhanced acoustic sensing. Top: the pressure field of sound is spatially compressed and amplified inside the high-refractive-index acoustic metamaterial before being detected by a sensor. Bottom: schematic metamaterial dispersion curve for acoustic waves with a high- k state. In such a metamaterial medium, sound propagation with a large wave vector k (measured by wave number) is enabled, rendering an effective high-refractive-index n eff = k z / k air . Full size image Analytical model of graded-index metamaterial waveguide The idea of enhancing acoustic sensing through pressure field amplification in the propagation medium stems from the strong wave compression effect in anisotropic high-refractive-index acoustic metamaterials, which cannot be achieved by using any natural materials whose acoustic refractive indices are lower than that of air. 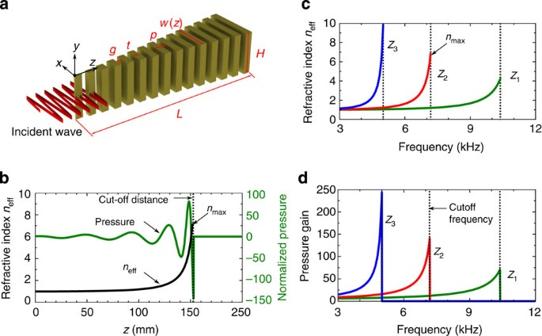Figure 2: Sound compression and pressure amplification effects in metamaterial based on analytical model. (a) Schematic of a tapered metamaterial slab comprised of an array of stainless plates spaced by air gaps with gap distanceg=1.4 mm and array periodicityp=3.4 mm. The height and thickness of plates areH=40 mm andt=2 mm, respectively. The widthwof each plate increases from 0.5 to 50 mm with a step of 0.5 mm. For simplicity, the metamaterial structure is considered as a 2D system and the propagation of acoustic wave is assumed to be confined in thex–zplane. (b) The wave compression effect in metamaterial. The spatial distribution ofneffand the spatial oscillation of normalized pressure field along the wave propagation direction are obtained by using equations (4) and (5) at 7.2 kHz, respectively. The pressure fields inside metamaterial region are normalized by the initial pressure amplitudeP(z=0) in equation (5), which is equal to the pressure amplitude of free-space incident wave. (c) Dispersion properties ofneffat different locations along the propagation axis (Z1=102 mm,Z2=153 mm andZ3=224 mm). (d) The corresponding pressure-gain spectra at different locations of the metamaterial. The pressure-gain spectrum at specific positionzin metamaterial is obtained asP(f,z)/P(f,z=0). Figure 2a illustrates a typical anisotropic acoustic metamaterial waveguide comprised of a periodic array of rectangular stainless steel plates spaced by air gaps. The width w of the steel plate is linearly changed, which renders a tapered metamaterial waveguide for guiding airborn acoustic waves ( Supplementary Note 1 ). To characterize the metamaterial response, the subwavelength array structure is regarded as a two-dimensional (2D) continuous, lossless acoustic medium with its effective mass density ρ x and ρ z , and bulk modulus B determined by the effective medium theory [23] as: Figure 2: Sound compression and pressure amplification effects in metamaterial based on analytical model. ( a ) Schematic of a tapered metamaterial slab comprised of an array of stainless plates spaced by air gaps with gap distance g =1.4 mm and array periodicity p =3.4 mm. The height and thickness of plates are H =40 mm and t =2 mm, respectively. The width w of each plate increases from 0.5 to 50 mm with a step of 0.5 mm. For simplicity, the metamaterial structure is considered as a 2D system and the propagation of acoustic wave is assumed to be confined in the x–z plane. ( b ) The wave compression effect in metamaterial. The spatial distribution of n eff and the spatial oscillation of normalized pressure field along the wave propagation direction are obtained by using equations (4) and (5) at 7.2 kHz, respectively. The pressure fields inside metamaterial region are normalized by the initial pressure amplitude P ( z =0) in equation (5), which is equal to the pressure amplitude of free-space incident wave. ( c ) Dispersion properties of n eff at different locations along the propagation axis ( Z 1 =102 mm, Z 2 =153 mm and Z 3 =224 mm). ( d ) The corresponding pressure-gain spectra at different locations of the metamaterial. The pressure-gain spectrum at specific position z in metamaterial is obtained as P ( f , z )/ P ( f , z =0). Full size image where F =( p − g )/ p is the filling ratio of steel plates in air, p is the periodicity of the array and g is the size of the air gap. ρ steel and B steel are the density and bulk modulus of steel material, respectively, and ρ air and B air are density and bulk modulus of air, respectively. With this simplified model, the local wave dispersion relation is obtained and further used to derive the effective refractive index of the metamaterial ( Supplementary Note 2 ), that is, Here, n air is the refractive index of air, f is the frequency of acoustic wave, z is the distance from the beginning of the tapered metamaterial waveguide ( z ≥0) and w ( z ) is the width of the metamaterial slab and it is assumed to be a continuous function along the propagation axis z . The highly anisotropic metamaterial structure with great difference between the effective density ρ x and ρ z enables propagation of acoustic waves with a large wave vector k z along the propagation direction ( Supplementary Note 3 ). As a result, a high effective refractive index much larger than that of the air ( n air =1) can be achieved, which overcomes the low-refractive-index limitation in natural acoustic materials. Here it should be noted that the effective index of the metamaterial is given as n eff = k z / k air , which describes the deviation of the wave vector from that of the air line ( k air is the wave vector in air) [42] , [43] . According to equation (4), the effective index n eff depends not only on the constant effective material parameters, but also on the geometric parameters of the metamaterial waveguide. Therefore, the effective refractive index can be readily tailored by engineering the geometric parameters. In this work, we consider a linearly tapered metamaterial device shown in Fig. 2a , which exhibits a graded refractive index (GRIN) distribution. As shown in Fig. 2b , when the GRIN metamaterial is used to guide a 7.2-kHz acoustic wave, n eff increases from 1 (air) to a larger value (for example, 7 at z =153 mm) along the propagation direction z . This indicates that the GRIN metamaterial waveguide can help not only achieve a high effective refractive index, but also overcome the wave vector and mode-field mismatch between the metamaterial waveguide and the background medium (air), thus enabling a high free-space (air) to metamaterial coupling efficiency ( Supplementary Note 5 ). Further, the closed-form pressure field in the metamaterial is obtained as ( Supplementary Note 4 ): This equation describes the spatial oscillation and spectral response of pressure field along the propagation axis ( x =0) of a GRIN metamaterial waveguide, which is governed by the spatial and spectral properties of n eff . On the basis of this equation, the pressure distribution along the propagation direction at a specific frequency (7.2 kHz) is obtained in Fig. 2b . It is evident that with the GRIN metamaterial, along the propagation direction, the wavelength gradually decreases and the wave pressure field is progressively growing, which renders a spatial compression of the acoustic wave along the propagation direction. Such a strong wave compression effect is the key to enable significant pressure field amplification (that is, pressure gain) in the metamaterial for enhancing acoustic sensing. Here it should be clarified that the ‘pressure gain’ of the passive metamaterial waveguide is different from the power gain of active devices. It is defined as the ratio of the acoustic pressure amplitude inside the metamaterial to that of the free-space incident waves ( Supplementary Note 6 ) [44] , [45] . Furthermore, the pressure field increases as n eff increases, with the highest pressure amplification achieved at the maximum n eff . However, n eff cannot be an arbitrarily large value. Note that the largest wave vector is determined as k z = π / p , which corresponds to the boundary of the first Brillouin zone in periodic systems [36] , [39] . The maximum effective refractive index n max is therefore determined as n max = k z / k air = c air /2 pf ( c air is the sound speed in air), which is limited by the periodicity p of the metamaterial structure. This introduces a spatial cutoff condition (that is, a cutoff distance along the wave propagation direction) and the propagation of acoustic waves is prohibited when n eff > n max (see Fig. 2b ). A similar cutoff behaviour can be observed in the frequency domain. In Fig. 2c,d , the dispersion property of n eff and the corresponding frequency response of the pressure gain at different locations of the metamaterial are shown, respectively. It can be seen that the pressure frequency response is determined by the local dispersion property of the refractive index (that is, n eff ( f )) and the pressure-gain spectrum manifests a unique asymmetric cutoff lineshape. This lineshape is distinctively different from the Lorentzian or Fano lineshapes that represent the characteristics of cavity resonance systems [46] . At the cutoff frequencies, the maximum refractive indices as well as maximum pressure gain can be achieved, while the acoustic waves are prohibited above these frequencies. Furthermore, the cutoff frequencies are found to be distinctive at different locations of the metamaterial, which renders the metamaterial the capability of frequency multiplexing. Numerical studies of GRIN metamaterial devices When acoustic waves propagate through small apertures and channels, the viscous and thermal losses can be significant, which is not taken into account in the analytical model. Here, we perform numerical thermoacoustic studies to characterize the acoustic response of practical metamaterial devices comprised of discrete subwavelength structures. 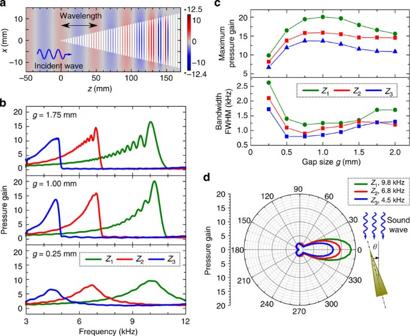Figure 3: Numerical studies of acoustic metamaterial waveguide. (a) FEM simulations of acoustic wave propagation in a 2D discrete metamaterial structure with an array of stainless plates spaced by air gaps. The distance between the air gaps is 1.4 mm and the array periodicity is 3.4 mm. The thickness of plates is 2 mm, and the width of each plate increases from 0.5 to 50 mm with a step of 0.5 mm. The incident acoustic wave is at 7.2 kHz. The pressure field distribution is normalized to the pressure amplitude of the free-space incident plane wave. The colour bar indicates the normalized pressure. (b) The pressure-gain spectra at different positions of the metamaterial for various gap sizes. Other geometric parameters are fixed. The positions (Z1,Z2andZ3) in the metamaterial structure are chosen to be consistent with those used inFig. 2. For the discrete metamaterial, the locationsZ1,Z2andZ3correspond to the centres of gaps 30, 45 and 66 counted from the beginning (z=0) of the tapered metamaterial waveguide, respectively. The pressure-gain spectrum at a specific gap position of the metamaterial is obtained as the pressure field in the gap centre normalized to that of the incident plane wave in the free space. (c) The maximum pressure gain (top) and pressure-gain bandwidth (bottom) with respect to various air gap sizesgobtained at different positions (Z1,Z2andZ3) of the metamaterials. The maximum pressure gain is obtained as the peak pressure gain inband the pressure-gain bandwidth is determined by using the full width at half maximum bandwidth of pressure-gain spectrum obtained inb. (d) The directivity patterns of the maximum pressure gain at different working frequencies. The pressure gains are obtained at positionsZ1,Z2andZ3(that is, gaps 30, 45 and 66), corresponding to the working frequencies at 9.8, 6.8 and 4.5 kHz, respectively. The inset shows the orientation of the metamaterial waveguide with respect to the direction of incident plane waves. Figure 3a shows the obtained pressure field distribution at a particular frequency (that is, 7.2 kHz corresponding to Fig. 2b ), where the wavelength of the pressure wave is shown to decrease and the pressure field is amplified along the propagation direction z . This result is consistent with the wave compression effect predicted by using the analytical model for continuous, lossless metamaterials, although a smaller pressure amplification (pressure amplification of ~12 compared with ~145 for the lossless metamaterial) is achieved due to the losses in the metamaterial. Due to the wave dissipation effect, the air gap size of the metamaterial structure is expected to be an important factor that affects the pressure amplification. Figure 3: Numerical studies of acoustic metamaterial waveguide. ( a ) FEM simulations of acoustic wave propagation in a 2D discrete metamaterial structure with an array of stainless plates spaced by air gaps. The distance between the air gaps is 1.4 mm and the array periodicity is 3.4 mm. The thickness of plates is 2 mm, and the width of each plate increases from 0.5 to 50 mm with a step of 0.5 mm. The incident acoustic wave is at 7.2 kHz. The pressure field distribution is normalized to the pressure amplitude of the free-space incident plane wave. The colour bar indicates the normalized pressure. ( b ) The pressure-gain spectra at different positions of the metamaterial for various gap sizes. Other geometric parameters are fixed. The positions ( Z 1 , Z 2 and Z 3 ) in the metamaterial structure are chosen to be consistent with those used in Fig. 2 . For the discrete metamaterial, the locations Z 1 , Z 2 and Z 3 correspond to the centres of gaps 30, 45 and 66 counted from the beginning ( z= 0) of the tapered metamaterial waveguide, respectively. The pressure-gain spectrum at a specific gap position of the metamaterial is obtained as the pressure field in the gap centre normalized to that of the incident plane wave in the free space. ( c ) The maximum pressure gain (top) and pressure-gain bandwidth (bottom) with respect to various air gap sizes g obtained at different positions ( Z 1 , Z 2 and Z 3 ) of the metamaterials. The maximum pressure gain is obtained as the peak pressure gain in b and the pressure-gain bandwidth is determined by using the full width at half maximum bandwidth of pressure-gain spectrum obtained in b . ( d ) The directivity patterns of the maximum pressure gain at different working frequencies. The pressure gains are obtained at positions Z 1 , Z 2 and Z 3 (that is, gaps 30, 45 and 66), corresponding to the working frequencies at 9.8, 6.8 and 4.5 kHz, respectively. The inset shows the orientation of the metamaterial waveguide with respect to the direction of incident plane waves. Full size image To further investigate the effect of losses, the pressure-gain spectra at various locations with respect to the air gap size are obtained in Fig. 3b . A trade-off effect on the pressure gain can be observed. First, decreasing the gap size results in an increase in the pressure gain, which qualitatively agrees with the analytical prediction (equation (5)) for lossless metamaterials. However, further narrowing the gap size leads to a decrease in the pressure gain, which cannot be predicted by the analytical model. This is believed to be the result of more significant dissipation due to the air viscous effect and thermal loss in smaller air channels. For the simulated metamaterial device, choosing a moderate gap width of 0.8–1.5 mm can help reach a good compromise between the pressure gain and wave propagation loss, and a significant pressure gain (10–20 times) can still be achieved ( Fig. 3c ). Furthermore, there is also a trade-off between pressure gain and bandwidth; as the gain increases, the bandwidth decreases (see Fig. 3c ). In addition, it is worth noting that other geometric parameters, such as the filling ratio of steel plates and tapering angle of the metamaterial waveguide, can also influence the pressure gain. It is expected that optimization of the metamaterial geometric parameters can lead to even better performance. For instance, increasing the taper angle can reduce the propagation distance of acoustic waves. This may decrease the thermoviscous dissipation, and thus improving the maximum achievable pressure gain in the metamaterial waveguide. On the other hand, an increase in the taper angle may cause more reflection and scattering losses of the acoustic waves propagating along the metamaterial waveguide, hence reducing the pressure gain in the metamaterial. Optimization of the geometric parameters is beyond the scope of this work. Interestingly, besides the pressure amplification, the metamaterial waveguide also exhibits a remarkable directional response. The directivity patterns of the maximum pressure gain of the metamaterial waveguide are obtained by using finite element method (FEM) simulations (see Fig. 3d ). It can be clearly seen that the maximum pressure gain is a function of the incident angle of the acoustic waves. It is also evident that at a 0° incident angle, the sound wave can be well coupled into the metamaterial waveguide and the highest pressure gain can be obtained, while at a 180° incident angle, the pressure gain is minimum due to the serious wave impedance mismatch at the air/metamaterial interface. The strong directional response of the metamaterial can be highly desirable in many acoustic sensing applications, for example, sound source localizations [47] , [48] , [49] . Experiments on metamaterial-enhanced acoustic sensing Taking the advantage of the pressure amplification effect offered by the metamaterials, the metamaterial-enhanced acoustic sensing system was developed. To measure the enhanced pressure fields inside the metamaterial, a miniature fibre optic microphone with a diameter of 323 μm was integrated with a fabricated GRIN metamaterial device, rendering a photonic–acoustic metamaterial hybrid sensing system, as shown in Fig. 4a . Since the size of the microphone is much smaller than the sound wavelength and the metamaterial unit cell, the wave propagation in the metamaterial structures will not be disturbed. The optical detection system is based on the low-coherence interferometer technique [8] (see Fig. 4a ). This hybrid sensing system has the advantages of both optical (for example, immunity to electromagnetic interferences, low noise, high sensitivity and so on) and acoustic metamaterial modalities (that is, pressure gain in the propagation medium and frequency multiplexing). 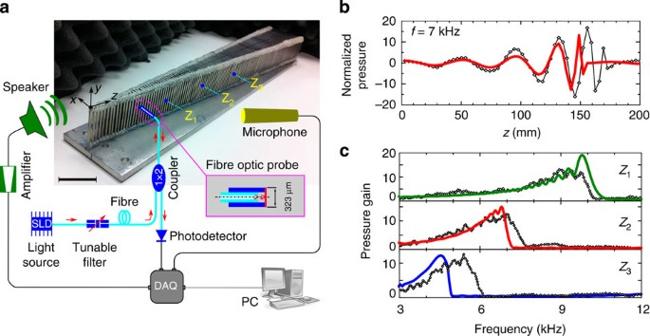Figure 4: Acoustic measurements of metamaterial response. (a) Schematic of photonic–acoustic metamaterial hybrid sensing system. The inset shows the configuration and dimension of the fibre optic probe. Scale bar, 40 mm. The metamaterial device was constructed with an array of stainless plates spaced by air gaps. The distance between the air gaps is 1.4 mm and the array periodicity is 3.4 mm. The height and thickness of plates are 40 and 2 mm, respectively. The width of each plate increases from 0.5 to 50 mm with a step of 0.5 mm. (b) Experimental characterization of wave propagation and compression in the metamaterial structure at 7 kHz. (c) Pressure-gain spectra measured at different gap positionsZ1,Z2andZ3, which correspond to gaps 30, 45 and 66 shown ina, respectively. Inb,c, the diamond dots represent the experimental data and solid lines represent the simulation results. Different colours of the simulation results correspond to different frequency bands. Figure 4: Acoustic measurements of metamaterial response. ( a ) Schematic of photonic–acoustic metamaterial hybrid sensing system. The inset shows the configuration and dimension of the fibre optic probe. Scale bar, 40 mm. The metamaterial device was constructed with an array of stainless plates spaced by air gaps. The distance between the air gaps is 1.4 mm and the array periodicity is 3.4 mm. The height and thickness of plates are 40 and 2 mm, respectively. The width of each plate increases from 0.5 to 50 mm with a step of 0.5 mm. ( b ) Experimental characterization of wave propagation and compression in the metamaterial structure at 7 kHz. ( c ) Pressure-gain spectra measured at different gap positions Z 1 , Z 2 and Z 3 , which correspond to gaps 30, 45 and 66 shown in a , respectively. In b , c , the diamond dots represent the experimental data and solid lines represent the simulation results. Different colours of the simulation results correspond to different frequency bands. Full size image By using the hybrid sensing system, we demonstrated the physical phenomena associated with wave compression and pressure-gain spectra in metamaterials predicted by using the analytical model ( Fig. 2b,d ). The experiments were conducted in an anechoic chamber, where acoustic plane waves generated from a speaker were coupled into the metamaterial device from the free space. The fibre optic probe was positioned at the centre of an air gap in the metamaterial. To study the wave propagation behaviour, we measured the phase and amplitude of the pressure field in each individual gap by scanning the fibre probe along the wave propagation direction, which was used to reconstruct the spatial pressure field oscillations in the metamaterial. In Fig. 4b , for instance, the reconstructed pressure field along the propagation direction for a 7-kHz incident acoustic wave is shown. This result clearly indicates that wave propagation in the discrete metamaterial structure behaves like that in a continuous medium. The phenomenon of wave compression and pressure amplification in the metamaterial was also well demonstrated, which is consistent with the theoretical prediction ( Fig. 2b ). The wave compression phenomena at other frequencies exhibit similar effects ( Supplementary Note 7 ; Supplementary Fig. 4 ). Further, the pressure-gain spectra at different gap positions in the metamaterial were obtained through frequency sweeping from 3 to 12 kHz. Representative pressure-gain spectra obtained at several gap positions are shown in Fig. 4c . More than tenfold pressure amplification is achieved. The lineshape of the spectra agrees well with those predicted by using the theoretical model and numerical simulations. The unique band-pass characteristic of the pressure-gain spectra of the metamaterial device may be exploited for acoustic frequency multiplexing applications. In addition, FEM simulations on a continuum-tapered metamaterial with anisotropic homogeneous material parameters determined by the effective medium model were performed. The simulation results are in good agreement with the experimental results, which also demonstrate the phenomena of wave compression and pressure amplification ( Supplementary Note 8 ). Overcoming the conventional acoustic detection limit Acoustic pulses are often used as transmission signals in acoustic communication, acoustic imaging and sonar systems. In these systems, the detection limit (that is, the minimum detectable pressure) is determined by the noise floor of the acoustic sensors. Here we demonstrated the feasibility of recovering weak acoustic pulse signals below the detection limit of a conventional acoustic sensing system by using a metamaterial-enhanced acoustic sensing system shown in Fig. 4a . In such a system, the pressure field (that is, acoustic signals) is compressed and amplified in the wave propagation medium (acoustic metamaterial) before being detected by a sensor. A series of Gaussian-modulated acoustic pulses (inset in Fig. 5a ) with a centre frequency of 9.3 kHz and a bandwidth of 0.5 kHz were generated from the speaker and used as acoustic input. The frequency and bandwidth of the acoustic pulses were chosen so that these pulses can be amplified in one of the pressure-gain bands of the metamaterial device (that is, position Z 1 in Fig. 4c ), where the fibre optic probe was positioned to detect the amplified acoustic field. The volume of the speaker was adjusted to control the signal-to-noise ratio (SNR) of the free-space acoustic signal measured by using the same fibre optic probe. As shown in Fig. 5a , the SNR achieved in the metamaterial is enhanced by more than 100 times (that is, >20 dB) compared with that obtained in the free space. Since the pressure detection limit is determined when SNR is 1, this SNR enhancement means that the detection limit of the metamaterial-enhanced sensing system is improved by over tenfold. This will enable the metamaterial-enhanced sensing system to detect weak acoustic signals below the detection limit of a conventional acoustic sensor (that is, SNR<1 in free space). In Fig. 5b,c , the measured time-domain and frequency-domain acoustic pulse signals in the free space are compared with those measured in the metamaterial. It can be seen that the measured free-space signal is completely overwhelmed by the noise (that is, SNR=0.27; Fig. 5b,c , top). This means that the free-space acoustic signal is smaller than the detection limit of the fibre optic probe. By contrast, owing to the strong field amplification effect in the metamaterial, the same weak acoustic pulse is successfully recovered (that is, SNR=32.7) in the metamaterial region with the fibre optic probe and the amplified pulse does not suffer from obvious distortions ( Fig. 5b,c , bottom). These results demonstrated that the metamaterial-enhanced sensing system can overcome the detection limit of a conventional acoustic sensor. 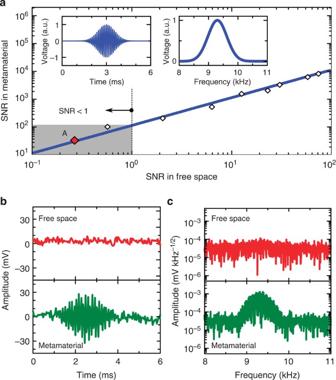Figure 5: Experimental demonstration of metamaterial-enhanced acoustic sensing. (a) SNR measured in the metamaterial compared with that obtained in free space. The input signal from the speaker was a series of Gaussian pulses with a centre frequency of 9.3 kHz and a bandwidth of 500 Hz. The inset shows the Gaussian pulse in time domain (left) and frequency domain (right). The diamond dots are the experimental data and the solid line is the fitted curve with a slope of 114, indicating about 20 dB SNR improvement by using the metamaterial-enhanced sensing system. In both free space and metamaterial, the SNR is calculated by using the total measured signal powerWin the frequency domain within the bandwidth of 9.05–9.55 kHz when the speaker was turned on compared with that obtained with the speaker turned off (W0, as noise floor), that is, SNR=(W−W0)/W0. In the grey highlighted zone, the measured free-space SNR is <1, indicating that the input signal is below the detection limit. (b,c) Time-domain and frequency-domain pulse signal measured in free space (top) and in the metamaterial (bottom). The SNR measured in the metamaterial device is 32.7 compared with the measured free-space SNR of 0.27, which corresponds to point A ina. Figure 5: Experimental demonstration of metamaterial-enhanced acoustic sensing. ( a ) SNR measured in the metamaterial compared with that obtained in free space. The input signal from the speaker was a series of Gaussian pulses with a centre frequency of 9.3 kHz and a bandwidth of 500 Hz. The inset shows the Gaussian pulse in time domain (left) and frequency domain (right). The diamond dots are the experimental data and the solid line is the fitted curve with a slope of 114, indicating about 20 dB SNR improvement by using the metamaterial-enhanced sensing system. In both free space and metamaterial, the SNR is calculated by using the total measured signal power W in the frequency domain within the bandwidth of 9.05–9.55 kHz when the speaker was turned on compared with that obtained with the speaker turned off ( W 0 , as noise floor), that is, SNR=( W−W 0 )/ W 0 . In the grey highlighted zone, the measured free-space SNR is <1, indicating that the input signal is below the detection limit. ( b , c ) Time-domain and frequency-domain pulse signal measured in free space (top) and in the metamaterial (bottom). The SNR measured in the metamaterial device is 32.7 compared with the measured free-space SNR of 0.27, which corresponds to point A in a . Full size image The essence of metamaterial-enhanced acoustic sensing technique is enabled by the unique wave compression and resulted pressure amplification effect in the GRIN metamaterials. Our proof-of-concept experimental results have demonstrated that these metamaterials can help improve the detection limit of current acoustic sensing systems by at least an order of magnitude. It should be noted that the metamaterial properties, such as spatial and spectral distributions of effective refractive index, can readily be designed by changing metamaterial geometric parameters such as the array periodicity, dimension and filling ratio of metal plates and waveguide tapering angle. This will allow unprecedented control of wave propagation and compression (for example, fast or slow compressions) and tailoring the pressure response spectrum (for example, narrowband or broadband) in metamaterials, which enables optimized metamaterial designs to further improve the performance of metamaterial-based sensing systems. Furthermore, the metamaterial-enhanced sensing technique has several unique features that distinguish it from other field-enhancement mechanisms, such as acoustic cavity resonance [44] or slow-wave antennas and waveguides [50] , [51] , [52] , [53] . Specifically, the strong asymmetric cutoff lineshape of the pressure spectrum in the metamaterial device is distinctively different from the response lineshapes of conventional acoustic cavities. The cavity resonance-based pressure field enhancement suffers from the bandwidth constraint due to the nature of its high-Q resonance, which can hardly satisfy the bandwidth requirements of many acoustic sensing systems. By contrast, the wave compression and resulting pressure field enhancement in the GRIN metamaterials is essentially a non-resonant process. The acoustic spectrum exhibits a high pressure gain and relatively broad working bandwidth. For example, the pressure-gain spectrum in the gap position Z 2 shown in Fig. 4c (middle) exhibits a 13-fold pressure amplification with a working bandwidth of 2.3 kHz. The broadband characteristic of our device also distinguishes it from the slow-wave antennas and waveguides that critically rely on the wave interference effect [50] and extremely low group velocities of guided waves [51] , [52] , [53] . These devices were usually designed to work at a single frequency (or within a narrow frequency band) corresponding to the band-edge region, and thus they are not suitable for broadband acoustic sensing applications. In addition, the pressure amplification mechanism of our device is also conceptually different from other broadband acoustic devices, such as exponential horns [54] and artificial cochleas [55] , which do not rely on the wave compression and pressure amplification effect enabled by the high-refractive-index acoustic metamaterials. It should be noted that the bandwidth of the metamaterial device can be further controlled by engineering n eff ( f ) (that is, dispersion of metamaterials). This will allow tailoring the lineshape of pressure-gain spectrum in metamaterials so that a narrower or wider gain bandwidth can be achieved. The metamaterial-enhanced sensing is thus promising for a broad area of applications, such as acoustic spectroscopy, frequency multiplexing for communications and sonar systems. Besides the pressure amplification, the GRIN metamaterial waveguides are also suitable for directional acoustic sensing. Since the pressure gain of the metamaterial device is found to strongly depend on the directions of incident waves, this phenomenon provides a physical basis for sound source localization using metamaterials, which can be useful for many acoustic sensing applications. In addition, in terms of device size, the width and height of the metamaterial devices can be designed to be subwavelength. The total length of the devices is determined by the wave compression distance, which can be just 2–4 wavelengths of the incident wave. This enables the development of compact metamaterial sensing devices, especially for sensing of ultrasonic waves that have much shorter wavelengths. On the other hand, integration of many individual metamaterial waveguides can enable a sensor array system (that is, metamaterial waveguide arrays), which is desirable for many acoustic sensing applications [56] . More interestingly, bulk acoustic metamaterials may be formed with strongly coupled metamaterial waveguide arrays [37] , [57] , which can provide numerous possibilities for large-scale acoustic wave manipulations. For instance, acoustic lens amplifiers may be realized, which can simultaneously implement wave focusing, compression and pressure amplification, thus enabling even greater signal enhancement that is beneficial for acoustic sensing and imaging systems. In conclusion, we have demonstrated the metamaterial-enhanced acoustic sensing, which has great potential to achieve performance and functionalities superior than the current acoustic sensing systems. We envision that the metamaterial-enhanced acoustic sensing can open up new possibilities to impact many fronts, including, but not limited to sonar systems, acoustic communication and navigation systems, noise source identification, non-destructive damage detection and medical imaging. Metamaterial sample preparation The metamaterial device was fabricated by assembling an array of 100 rectangular stainless steel plates, which were made by using the laser cutting technique. The thickness t and height H of plates are 2 and 40 mm, respectively. The width of each plate w increases from 0.5 to 50 mm with a step of 0.5 mm. The steel plates, from big to small, were stacked with plastic spacers (with a dimension of 2 mm × 2 mm × 1.4 mm) attached to the corners of each plate. Fabrication of optical fibre acoustic probe The miniature optical fibre acoustic probe was constructed by using a graphene diaphragm as the pressure sensing transducer, a glass capillary tubing and a single-mode fibre. The graphene diaphragm was chosen to achieve high pressure sensitivity and large bandwidth simultaneously. A commercially available graphene film was floated on water surface and then lifted onto a glass capillary tube (Polymicro TSP150375) with an inner diameter of 150 μm and outer diameter of 323 μm. The film was firmly adhered to the cavity surface due to the van der Waals force. A single-mode fibre was then inserted into the capillary tube from the other end. The distance between the fibre endface and graphene film was adjusted to be 60 μm, which was achieved by monitoring the interference spectrum with a white-light interferometry system. A Fabry–Pérot cavity was thus formed between the fibre endface and the graphene film, whose cavity length changes with respect to the external acoustic pressure field. Experimental setup and measurements Experiments were conducted under room temperature inside a customized anechoic chamber to isolate the environmental noise. A loudspeaker (ESS, model Heil AMT) was placed 2 m away in front of the tapered end of the metamaterial device, which was used to generate plane acoustic waves incident from air into the metamaterial region. The pressure in the metamaterial was measured using the fibre optic probe in a low-coherence fibre optic interferometry configuration. The low-coherence fibre optic interferometer system (see Fig. 4a ) consists of a super-luminescent diode (Thorlabs, Model S5FC1018S), the fibre optic probe serving as a sensing interferometer, a Fabry–Pérot tunable filter (Micro Optics, FFP-TF2) used as a read-out interferometer and a photodetector (New Focus, Model 2011). By using the fibre optic probe, the phase and amplitude of pressure fields were measured in each gap along the propagation axis of the metamaterial. To obtain the phase of the pressure fields in the metamaterial, a condenser microphone (Brüel & Kjær, Type 2669) was placed in front of the speaker to determine the original phase of the pressure field in free space. The measured data were recorded by using a PC via a data acquisition card (DAQ, National Instruments USB-6259) for further processing. To obtain the pressure-gain spectrum, the pressure responses at various specific gap positions in the metamaterial are measured by frequency sweeping from 3 to 12 kHz with a resolution of 20 Hz, and the results are normalized to those measured in the free space. Numerical calculations FEM simulations of acoustic wave propagation in metamaterial structures were carried by using thermoacoustic module in COMSOL Multiphysics V4.4, which takes into consideration the viscous and thermal losses for acoustic wave propagation. Due to the high density and Young’s modulus of steel relative to the air, the sound waves can hardly penetrate into the steel material, and thus the stainless steel plates in the metamaterial can be treated as rigid bodies. In the FEM simulations, the steel–air interfaces are described by using Neumann boundary conditions. A plane wave radiation boundary condition was used to simulate the incident sound waves, and perfect matched layers were added on the outer sidewalls to prevent reflected acoustic waves from the boundaries. The mesh element size was set to be smaller than 1/15 of the smallest simulated wavelength. To improve the simulation accuracy, finer boundary layer meshes were applied to the domains adjacent to the boundaries of steel plates, which can help capture the viscous and thermal dissipations due to the sound–plate interactions in metamaterial structures. How to cite this article: Chen, Y. et al. Enhanced acoustic sensing through wave compression and pressure amplification in anisotropic metamaterials. Nat. Commun. 5:5247 doi: 10.1038/ncomms6247 (2014).